Variation in genomic landscape of clear cell renal cell carcinoma across Europe The incidence of renal cell carcinoma (RCC) is increasing worldwide, and its prevalence is particularly high in some parts of Central Europe. Here we undertake whole-genome and transcriptome sequencing of clear cell RCC (ccRCC), the most common form of the disease, in patients from four different European countries with contrasting disease incidence to explore the underlying genomic architecture of RCC. Our findings support previous reports on frequent aberrations in the epigenetic machinery and PI3K/mTOR signalling, and uncover novel pathways and genes affected by recurrent mutations and abnormal transcriptome patterns including focal adhesion, components of extracellular matrix (ECM) and genes encoding FAT cadherins. Furthermore, a large majority of patients from Romania have an unexpected high frequency of A:T>T:A transversions, consistent with exposure to aristolochic acid (AA). These results show that the processes underlying ccRCC tumorigenesis may vary in different populations and suggest that AA may be an important ccRCC carcinogen in Romania, a finding with major public health implications. Renal cancer is diagnosed in more than 330,000 people each year worldwide, and accounts for 2.4% of all adult cancers and over 140,000 deaths annually [1] . Incidence rates have been increasing sharply with unexplained variation in different countries. The highest rates that are observed worldwide occur in Central Europe [2] , and in particular in the Czech Republic, reaching 24.1/100,000 in men and 10.5/100,000 in women (world population age-standardized rates), while the equivalent figures for the United Kingdom are 10.9/100,000 and 5.8/100,000. Approximately 90% of renal cancers are renal cell carcinomas (RCCs) that develop in the renal parenchyma [2] , with conventional (clear cell) RCC (ccRCC) being the most common (70–80%) histological type. Somatic mutations or epigenetic alterations of the von Hippel–Lindau tumour suppressor gene ( VHL ) are observed in >80% of ccRCC [3] , [4] . A modest proportion (2–4%) of RCC is associated with VHL syndrome caused by germline mutations in VHL [5] . Results from genome-wide association studies have identified common germline variants associated with increased susceptibility for developing ccRCC [6] , [7] , and recent sequencing efforts have revealed recurrent somatic mutations in a number of genes including PBRM1 , SETD2 and BAP1 (ref. 8 ). Recognized environmental and lifestyle risk factors for RCC include tobacco smoking, excess body weight and hypertension, as well as a history of chronic kidney diseases [2] , [9] . Previously somatic mutation patterns in patients from different European populations have not been systematically examined. Here we present the results of a whole-genome sequencing (WGS) study of ccRCC patients from four European countries (Czech Republic, United Kingdom, Romania and Russia), and we identify a specific mutational pattern that is predominant in the patients from Romania but not elsewhere. In addition to the WGS analysis of somatic variations, we also present results from a genome-wide transcriptome analysis in a subset of the study samples. 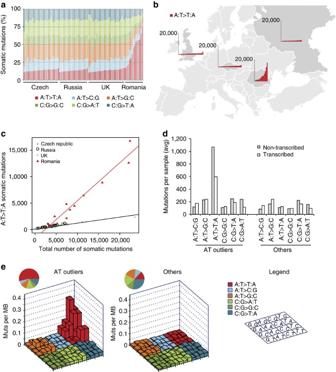Figure 1: Single-base substitution patterns in 94 ccRCC samples. (a) Proportion of observations within different base substitution classes for each ccRCC sample pair. (b) Number of A:T>T:A transversions in samples from the four countries included in the study. (c) The number of A:T>T:A transversions plotted against the total number of mutations in each sample. The graph also shows the linear regression lines for Romanian samples (red) and other samples (black). (d) Frequencies of six base substitution classes in Romanian outliers and other samples for somatic mutations within genes categorized into non-transcribed and transcribed strands. A:T>T:A transversions occur preferentially on the non-transcribed strand in the Romanian outliers. (e) Lego plot showing the number of somatic mutations with the surrounding sequence context for the Romanian outliers and other sample pairs. The plot illustrates the preference for A:T>T:A transversions within the context C/T[A:T]A/G, but also the overall increased frequency of A:T>T:A and increases of other mutational classes for the Romanian outliers. Molecular profiling of the clinical cohort Table 1 and Supplementary Data 1 provide summary and individual-level data on patients. We undertook a comprehensive molecular evaluation of the samples using WGS, single-nucleotide polymorphism (SNP) arrays (Illumina Human660-Quad BeadChip) and transcriptomics (RNA-seq). Matched tumour and blood DNA samples were available on 94 of the study participants, and WGS was made to an average depth of 54 × coverage in all of these samples ( Supplementary Data 2 ). We observed >99% concordance between SNP genotypes and sequence-based single-nucleotide variation (SNV) at the same sites in all 86 pairs with both data, attesting to the accuracy of the sequence calls. RNA from tumours was available for 92 patients (63 with WGS data), and from matched normal adjacent tissue for 45 of these (36 with WGS). We obtained an average of 81 million reads per sample from the RNA-Seq data, of which 90% were retained for further analysis based on the mapping results, the vast majority (94.0%) of which localized to protein coding genes. Table 1 Characteristics of the patients in the study. Full size table Genome sequencing results We detected 4,904 somatic mutations on average per sample pair corresponding to a mean of 1.79 somatic mutations per Mb after correcting for regions with low coverage (see Methods). Intergenic regions were seen to have higher mutation rates (2.02 Mb −1 ) than other genome regions ( Supplementary Fig. 1 ). Notably, the overall somatic mutation rate in coding regions was significantly less than this (1.54 Mb −1 , rate ratio=0.76, 95% confidence interval 0.74–0.79) corroborating previous literature [10] . Similarly, other regions associated with genes (for example, 5′ untranslated region (UTR), 3′UTR and introns) had lower rates than intergenic regions as shown in Supplementary Fig. 1 . Regions corresponding to DNaseI hypersensitive (DHS) sites (see Methods for definition) also had a lower overall somatic mutation rate (1.66 Mb −1 ) when compared with intergenic regions (rate ratio =0.82, 95% confidence interval 0.81–0.83) in concordance with a recent report in other cancers [11] . We did not detect significant patterns of recurrent mutations in non-coding regions of the genome (see below for coding regions). We identified loss-of-heterozygozity and other copy number variants (CNVs) at 1,008 sites (with sizes ranging from 450 kb to 197.7 Mb and between 0 and 48 CNV differences per pair; Supplementary Data 3 ) and we found 1,418 additional putative structural rearrangements ( Supplementary Data 4 ) with further analyses as described (Methods). Among recurrently affected loci, loss of chromosome 3p, the most frequent CNV, was observed in 90% of samples, whereas loss of all of chromosome X was observed in 7.4% of samples ( Supplementary Fig. 2 ), which is a novel recurrent aberration that has not previously been reported in ccRCC. A geographic specific mutational signature We observed different somatic mutation frequencies associated with patient country-of-residence (Kruskal–Wallis P =0.003; see Fig. 1 ). This was principally due to A:T>T:A transversions, which were found to be strikingly elevated in some tumours ( Fig. 1a,b ). We analysed the SNV patterns to identify such outlier samples as described in the Methods. Twelve sample pairs, all from Romania, accounted for the significantly increased A:T>T:A transversion rate ( Fig. 1c and see also Supplementary Data 2 and Supplementary Fig. 3a ). One additional Romanian sample pair (RO6) was a potential A:T>T:A outlier, while only one Romanian sample pair (RO12) exhibited no evidence of such a deviation. In the 12 outliers from Romania, the overall rates of somatic mutations were substantially higher than elsewhere (4.01 Mb −1 versus 1.48 Mb −1 ) and A:T>T:A transversions comprised 21–74% of all the somatic mutations detected ( Fig. 1a ). After removal of A:T>T:A, the pattern of mutations in other SNV classes remained slightly higher in the outliers compared with other samples ( Supplementary Fig. 3b , Kruskal–Wallis P =0.046). Country-of-origin was not significantly correlated to mutation counts when the Romanian sample pairs were excluded from the analysis (Kruskal–Wallis, P =0.10). Figure 1: Single-base substitution patterns in 94 ccRCC samples. ( a ) Proportion of observations within different base substitution classes for each ccRCC sample pair. ( b ) Number of A:T>T:A transversions in samples from the four countries included in the study. ( c ) The number of A:T>T:A transversions plotted against the total number of mutations in each sample. The graph also shows the linear regression lines for Romanian samples (red) and other samples (black). ( d ) Frequencies of six base substitution classes in Romanian outliers and other samples for somatic mutations within genes categorized into non-transcribed and transcribed strands. A:T>T:A transversions occur preferentially on the non-transcribed strand in the Romanian outliers. ( e ) Lego plot showing the number of somatic mutations with the surrounding sequence context for the Romanian outliers and other sample pairs. The plot illustrates the preference for A:T>T:A transversions within the context C/T[A:T]A/G, but also the overall increased frequency of A:T>T:A and increases of other mutational classes for the Romanian outliers. Full size image In the Romanian outliers, we observed a preference for A:T>T:A to occur within the specific sequence context of C/T[A:T]A/G ( Fig. 1e and Supplementary Fig. 3c,d ). This pattern accounted for 50% of A:T>T:A transversions in outliers compared with 26% in other samples. However, A:T>T:A was more frequent in the outliers irrespective of the context ( Supplementary Fig. 3d ). Finally, we observed a strong bias for a location on the non-transcribed strand for A:T>T:A transversions within genes in the Romanian outliers ( Fig. 1d ). Exposure to aristolochic acid (AA) is known to produce an increased frequency of A>T mutations with such strand bias [12] and has previously been shown to lead to AA nephropathy (AAN) characterized by chronic renal disease and to rare transitional cell carcinomas of the upper urinary tract [13] , [14] , but has not been reported as an environmental risk factor in ccRCC. Other mutational patterns One UK sample pair (UK24) with a very high somatic mutation rate (7.61 Mb −1 ) exhibited a relative predominance of A:T>G:C and C:G>A:T mutations ( Supplementary Fig. 4 ). This was the only obvious outlier with a potential unique mutational pattern outside of the Romanian sample pairs. We eliminated UK24 and all the Romanian sample pairs to conduct further analyses of the somatic mutation patterns. We found that the total number of somatic mutations increased significantly with the patients’ age (Pearson r 2 =0.3; P =2 × 10 −5 ; Supplementary Fig. 5a ). This observation included C>T mutations in the context of CpG dinucleotides, as reported previously in ccRCC and other cancers [15] , [16] , but it held equally for all other SNV classes ( Supplementary Fig. 5b ). Somatic mutations in genes We identified genes that harboured non-silent somatic mutations with a frequency significantly greater than background rates ( P <0.05 from MuSiC [17] ), or with non-silent somatic mutations seen in at least two patients. These mutations were further filtered by in silico analyses and subject to verification by an orthogonal sequencing method resulting in 1,239 validated mutations out of 1,317 that could be tested (94.1%; see Methods for details). Among tested mutations, 200 were indels from which 187 (93.5%) were validated and 1,117 were nucleotide substitutions from which 1052 (94.2%) were validated. The filtering and validation procedures led to a list of 583 genes ( Supplementary Data 5 ). Non-silent A:T>T:A substitutions were more frequent in the Romanian outliers compared with other patients (38% versus 11%; P <10 −33 ); however, only 9 of the 583 genes were in the list uniquely because of A:T>T:A substitutions in these patients (see Supplementary Data 6 for further information on non-silent A:T>T:A mutations). After removal of the Romanian sample pairs, the number of genes harbouring non-silent mutations did not significantly vary with country-of-residence (Kruskal–Wallis, P =0.08). We found a significant association between number of non-silent mutations and the patients’ age (Pearson r 2 =0.46; P =5 × 10 −7 with Romanian pairs excluded; Supplementary Fig. 5c ) that was stronger than that in the WGS data overall. 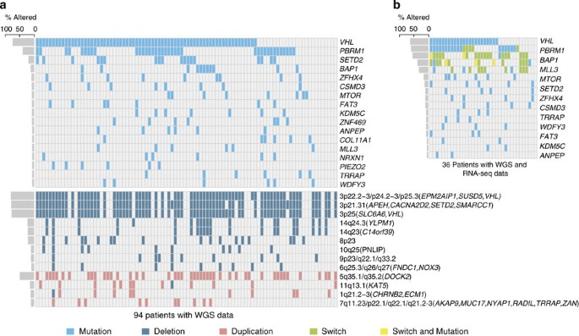Figure 2: Patterns of somatic variations in ccRCC samples. Left histograms show percentages of affected samples. (a) Upper heat map, somatic mutations; bottom heat map, copy number losses (blue) and gains (red) in 94 samples with sequencing data. Affected genes in each locus that harbour somatic SNVs are listed in the parentheses. (b) Patient-specific mutation and switch events affecting most frequently mutated genes (shown ina) detected in the 36 samples paired samples with both genomic and RNA analysis. The most frequently mutated genes are shown in Table 2 and Fig. 2 . The prevalence of VHL mutations in our patients (73%) is similar to that reported in our previous studies (70–80%) [3] , [4] but substantially higher than those found in recent next-generation sequencing studies of ccRCC, which have reported VHL mutations in 27% (ref. 18 ), 40% (ref. 19 ), 52% (ref. 20 ) and 55% (ref. 21 ) of samples. Although some of the variation may be due to ethnic origin, patient selection, pathology review criteria and/or sample tumour cell content, false-negative next-generation sequencing results have been evoked as a factor affecting previous studies [20] . VHL was mutated in 8 of the 12 Romanian outlier; however, none of these mutations were A:T>T:A transversion. In one patient, we identified a germline mutation (missense) in VHL of unknown functional significance. Table 2 Frequency of events for principal genes and pathways harbouring non-silent somatic variants. Full size table Figure 2: Patterns of somatic variations in ccRCC samples. Left histograms show percentages of affected samples. ( a ) Upper heat map, somatic mutations; bottom heat map, copy number losses (blue) and gains (red) in 94 samples with sequencing data. Affected genes in each locus that harbour somatic SNVs are listed in the parentheses. ( b ) Patient-specific mutation and switch events affecting most frequently mutated genes (shown in a ) detected in the 36 samples paired samples with both genomic and RNA analysis. Full size image Additional known ccRCC genes mutated in our cohort include PBRM1 (39%), SETD2 (19%), BAP1 (12%) and KDM5C (7%). No A:T>T:A mutations were found in SETD2 , BAP1 or KDM5C in Romanian outliers (see below for PBRM1 ). In addition to PBRM1 , genes encoding members of the SWI/SNF complex were mutated in 55% of ccRCCs studied here. Taking histone modifier genes into account, we found that 80% of the series was affected by mutations in epigenetic regulator pathways ( Supplementary Fig. 6 ). Novel genes with recurrent mutations in our data include FAT3 (7%), WDFY3 (6%) and ANPEP (6%) as shown in Table 2 . In addition to FAT3 , somatic mutations were also identified in other genes encoding Fat cadherins including FAT1 , FAT2 and FAT4 accounting for 20% of the subjects included in this study. We performed additional analysis across all genes but did not find any recurrent mutation in the promoters, UTRs or introns, nor in other regions (for example, DHS regions). Interestingly, PBRM1 was mutated in 10/12 (83%) of Romanian outliers compared with 27/82 (33%) in other sample pairs ( P =0.001), but only three of the mutations in the outlier group have the characteristic transversion pattern discussed above. This observation led us to further examine the overall relationship of somatic mutation frequencies with PBRM1 mutations. Because of the predominance of A:T>T:A mutations in PBRM1 mutated patients in Romania, we initially removed these transversions from consideration. We found that the presence of non-silent PBRM1 mutations was associated with higher overall mutation rates in the other mutation classes (Kruskal–Wallis, P =0.002). When we excluded the Romanian and UK outlier samples, but this time included A:T>T:A in the analysis, we again found a significant association (Kruskal–Wallis, P =0.009). However, we saw similar but nonsignificant trends for the other frequently mutated genes, where there may be lower power to detect an association because of the relative numbers of mutated and non-mutated sample pairs; thus, the PBRM1 observation may simply be due to association of higher somatic mutation rates genome wide with increased mutation frequencies in all the principal driver genes. Analysis of the relationship between clinical variables and the presence or absence of somatic mutations in genes with a mutation frequency of >10% identified significant associations only of both PBRM1 mutations ( P =0.043) and SETD2 mutations ( P =0.014) with higher-stage tumours ( Supplementary Fig. 7 ). As tumour stage is defined by local invasiveness (T), lymphatic infiltration and growth in lymph node (N) and metastasis (M), we also examined these variables. PBRM1 mutations only were associated with T ( P =0.05) but other variables and genes showed no significant relationships. Differential gene expression and differential splicing We found that 12,849 protein-coding genes (60% of genes annotated as such in Ensembl 66) were expressed on average at 1 fragments per kilo bases of exons for per million mapped reads (FPKM) or more in either the panel of 91 tumour samples, or in the 45 normal samples. In a paired analysis using only 45 samples with RNA-Seq data from matched tumour and adjacent normal tissue, we detected 3,272 protein-coding genes that were differentially expressed with more than twofold change between tumour and normal (false discovery rate (FDR)<0.01; Supplementary Data 7 and 8 ; see also Methods). Hierarchical clustering did not reveal any subgroups with correlations with clinical variables (results not shown). Expression data in paired samples were available for only two of the Romanian patients and in tumour only for three additional patients, which precluded an analysis of the subset with frequent A:T>T:A mutations. Individual genes were then examined for statistically significant differences in the levels of exon usage in the 45 matched tumour and adjacent normal samples, a metric that can be used as an indicator of differential splicing (see Methods). We detected 7,842 genes (7,182 protein coding) that manifested significant differences for at least one exon (with FDR<0.01; Supplementary Data 9 ). On the other hand, from transcript-centric analysis, we found that the average number of expressed transcripts per gene was higher in tumours compared with normal samples ( Supplementary Fig. 8 ). Transcript expression levels were also more variable in tumours compared with normal samples ( Supplementary Fig. 8 ), and such variability was correlated with the number of annotated transcripts (Pearson r 2 =0.75; P <0.001). Consistent with previous observations [22] , we observed gene expression to be dominated by one transcript in most cases, both in tumours and normal samples ( Supplementary Fig. 9 ). However, the number of genes with a dominant transcript was significantly different between tumour and normal samples ( P <0.001; Methods). When focusing on the most abundant transcript within each gene (major transcript), 50% of the genes with altered splicing were predicted to change major transcripts between the normal and tumour in at least one sample pair (referred to as switch events; Fig. 3 ). However, when applying additional filtering to require at least twofold or fivefold difference between the first and second most abundant transcripts, the number of such switch events was reduced to 25% and 2% of the genes, respectively, most of which were observed in a small number of samples ( Fig. 3b ). 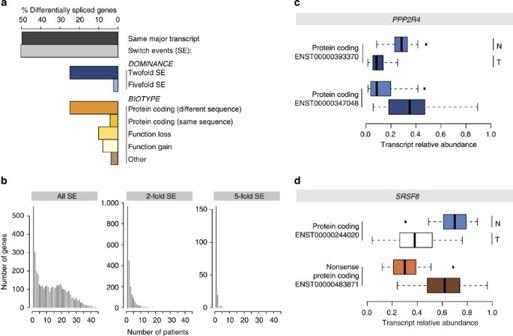Figure 3: Switch events in 45 matched normal and tumour samples. (a) Frequencies of different categories of switch events. (b) Number of patient sample pairs affected by switch events in different categories. (c,d) Box plots showing median, upper and lower quartiles of transcript relative abundance forPP2R4andSRSF6. Figure 3c,d provide examples of switch events in PP2R4 and SRSF6 , respectively, and show that a possible loss of function can occur through changes in the dominant transcript isoform even when no significant differential expression is observed on a gene level (see Supplementary Notes for details). Taken together, these findings indicate that extreme splicing changes are mostly non-recurrent, and suggest that splicing variation in ccRCC principally affects lower abundance transcripts. Figure 3: Switch events in 45 matched normal and tumour samples. ( a ) Frequencies of different categories of switch events. ( b ) Number of patient sample pairs affected by switch events in different categories. ( c , d ) Box plots showing median, upper and lower quartiles of transcript relative abundance for PP2R4 and SRSF6 . Full size image Modified expression for somatically mutated genes Of the 583 genes with non-silent somatic mutations, 104 (18%) also exhibited differential expression ( Supplementary Data 7 and 8 ) and 91 (15%) were observed to have switch events (using a twofold difference criterion and required observation in at least two patients; Supplementary Data 10 ). We evaluated the possible effect that mutation status might have on transcript expression levels by considering differences in transcript abundance for the 32 most frequently mutated genes. The results are shown in Supplementary Data 11 . We categorized tumours according to mutation status (nonsense/frame-shift, missense and no mutation) and also compared with transcript abundance in normal tissue. SETD2 exhibited nominally significant differences between mutation classes with tumours in the class of nonsense/frame-shift mutations had lower average expression ( Supplementary Fig. 10 ). We also found marginally significant results for ZFHX4 . However, neither result remained significant after adjustment for multiple testing. Interestingly, VHL exhibited no switch events, while PBRM1 , the second most frequently mutated gene, was affected by switch events in 5 of the 36 patients tested, none of whom harboured somatic mutations in this gene. Other mutated genes recurrently affected by switch events included BAP1 , PTEN and MTOR affected by switch events in 20.2%, 6.4% and 9.6% of the studied samples, respectively ( Fig. 2b and Supplementary Fig. 11 ). MLL3 , a histone methyltransferase involved in transcriptional activation, also emerged as an interesting example, as it was mutated in 6% of tumours in our data, and was affected by switch events in an additional 9.5%. Similarly, the transcription factor ETS1 was mutated in only one patient but was widely affected by switch events and expression changes ( Supplementary Fig. 12 ). This is consistent with previous reports that point to a disruption of expression levels for this gene in ccRCC [23] . Switch events affecting other recurrently mutated genes and genes involved in cellular processes associated with renal cancer are depicted in Supplementary Figs 11 and 12 , and discussed in the Supplementary Notes . The occurrence of switch events and somatic mutations in the same gene and patient were not mutually exclusive ( Supplementary Data 12 ). Identification of fusion genes Following in silico screening (see Methods) and validation by reverse transcription–PCR, we identified six tumour-specific fusion events ( Table 3 , Fig. 4 and Supplementary Fig. 13 ). Two fusion partner genes ( MED15 and TFE3 ) shown in Fig. 4 participate in the TGFβ/SMAD pathway, known to play a role in renal cancer development [24] , while 9 out of the 12 fusion partners ( CWC25 , CGNL1, SH2D3C , RAB31 , LRSAM1 , MED15 , SLC12A4 , TFE3 and TCF12 ) code for phosphoproteins, which are known with important roles in signalling pathways [25] . All the confirmed chimeras appeared to be associated with inversion, as the fusion partner genes were located on opposite strands. Further details about fusion events are provided in the Supplementary Notes . Table 3 Tumour-specific fusion events. 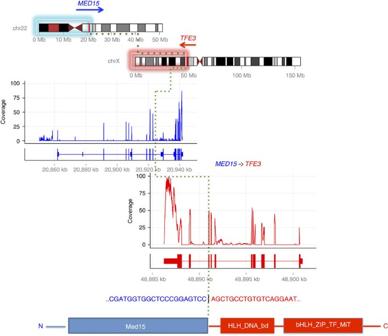Figure 4: Schematic representation of theMED15->TFE3fusion event. The figure shows the chromosome ideograms, transcript structures and number of reads mapping to the two partner genes. The dashed green line indicates the fusion breakpoint. The retained protein domains are shown at the bottom of the figure. Full size table Figure 4: Schematic representation of the MED15 -> TFE3 fusion event. The figure shows the chromosome ideograms, transcript structures and number of reads mapping to the two partner genes. The dashed green line indicates the fusion breakpoint. The retained protein domains are shown at the bottom of the figure. Full size image Pathway analysis Using the Kyoto Encyclopedia of Genes and Genomes (KEGG) data sets, we performed pathway analysis for genes affected by somatic mutations or transcriptome alterations (see Methods). Pathway analysis of the 583 genes harbouring somatic mutations showed significant enrichment for focal adhesion and phosphatidylinositide 3-kinase (PI3K) pathways (FDR=5 × 10 −07 and FDR=0.003, respectively; Supplementary Data 13 ). Overall, 59% of tumours in our study showed non-silent somatic mutations in one or more of 32 genes from these two pathways ( Table 2 ). Recurrent mutations in constituents of PI3K–mammalian target of rapamycin (mTOR) signalling have recently been reported in ccRCC [19] , [20] . We observed non-silent somatic mutations or CNVs at each of PIK3R1 , PTEN and MTOR in >5% of tumours and somatic variations at lower frequencies in other genes involved in PI3K–mTOR signalling. The Focal adhesion pathway contains genes that act upstream of PI3K (and of the FAK and Src pathways). We observed frequent somatic variations in genes encoding extracellular matrix (ECM) molecules, integrin receptors, members of the collagen family and genes coding for laminin chains in addition to genes coding for receptor tyrosine kinases ( Supplementary Data 14 and Fig. 5 ). 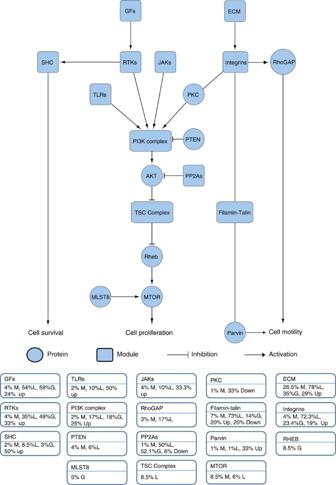Figure 5: Somatic variants in the focal adhesion and PI3K pathways identified in the ccRCC patients from our study. This figure shows interactions of the focal adhesion and PI3K pathway modules (adapted from KEGG). GFs, growth factors; ECM, extracellular matrix; RTKs, receptor tyrosine kinases; TLRs, Toll-like receptors; Jaks, janus kinases; PKC, protein kinase C; PP2As, Ser/Thr protein phosphotase 2A subunits; M, mutated; L, copy number loss; G, copy number gain; Up, upregulated; Down, downregulated; %, percentage of affected patients for M, L and G, and percentage of affected genes within each module for Up and Down fromSupplementary Data 14. Figure 5: Somatic variants in the focal adhesion and PI3K pathways identified in the ccRCC patients from our study. This figure shows interactions of the focal adhesion and PI3K pathway modules (adapted from KEGG). GFs, growth factors; ECM, extracellular matrix; RTKs, receptor tyrosine kinases; TLRs, Toll-like receptors; Jaks, janus kinases; PKC, protein kinase C; PP2As, Ser/Thr protein phosphotase 2A subunits; M, mutated; L, copy number loss; G, copy number gain; Up, upregulated; Down, downregulated; %, percentage of affected patients for M, L and G, and percentage of affected genes within each module for Up and Down from Supplementary Data 14 . Full size image Among downregulated genes, we observed highly significant (FDR<10 −9 ) enrichment in pathways involved in energy metabolism such as oxidative phosphorylation, known to be frequently impaired in ccRCC cells as part of a general metabolic shift [26] , carbon metabolism, the citrate cycle and amino acid metabolism ( Supplementary Data 15 ). Among key pathways enriched for upregulated genes were cytokine–cytokine receptor interaction, cell adhesion molecules and the chemokine signalling. Focal adhesion and PI3K pathways were also enriched for upregulated genes (FDR=2 × 10 −5 and FDR=2 × 10 −8 , respectively; Supplementary Data 16 ). ‘Metabolic pathways’ was the only KEGG pathway that showed evidence of enrichment for genes involved in switch events (using the criteria of a twofold expression difference seen in at least two patients). However, the protein processing in endoplasmic reticulum and mTOR signalling pathways also showed some evidence of enrichment ( P =0.001 without multiple testing correction, FDR=0.14; Supplementary Data 17 ). The latter is relevant in the context of PI3K-Akt and focal adhesion. Collectively, these results show that focal adhesion–PI3K–mTOR molecular axis is recurrently affected by somatic mutations and/or abnormal gene expression patterns in ccRCC ( Supplementary Data 14 and Fig. 5 ). A high rate of A:T>T:A transversions, as seen in the large majority of our Romanian samples, has not previously been reported in ccRCC. The predominance of A>T transversion on the non-transcribed strand of DNA along with a preference for deoxyadenosine in the C/T[A:T]A/G motif supports exposure to AA as the underlying factor. Similar patterns have recently been observed in urothelial carcinoma of the upper urinary tract in patients [12] , [27] as well as in cultured primary cells [27] , [28] exposed to AA, with C/T[A:T]G being the preferential sequence context. Our WGS data show that a less marked increase in A>T transversions also occurs in other sequence contexts. According to GLOBOCAN data, Romania is in the lower range of annual kidney cancer incidence rates, with 8.19 new cases per 100,000 in men and 3.71 per 100,000 in women (world population age-standardized rates). However, GLOBOCAN estimates for Romania are largely based on the regional registry that is located in the northwest part of the country (far from the area where cases were recruited for this study) as well as registries of neighbouring countries (Bulgaria and Slovakia) [29] . In 2007, The Romanian Ministry of Health initiated additional regional cancer registries but these are not yet fully functional and several more years will be needed to accurately map kidney cancer incidence across Romania to evaluate whether there are regional disparities that could be due to lifestyle habits. In parts of Asia, AAN occurs through widespread use of AA-containing herbal remedies [30] . In Europe, this practice has not been commonly reported and the use of Aristolochia fangchi in slimming regimen—which first triggered the attention to the associated risk of urothelial cancer in Belgium women [14] —appeared to be unintentional. Balkan endemic nephropathy (BEN) is thought to be due to the ingestion of wheat flour contaminated with seeds of Aristolochia clematitis [31] . BEN has been described as affecting people of the alluvial plains along the tributaries of the Danube River in Croatia, Bosnia and Herzegovina, Serbia, Bulgaria and Romania [31] . Interestingly, the catchment area of the Bucharest hospital where cases were recruited does not cover the Romanian population of the BEN area, who are usually hospitalized in Timisoara or Craiova, in the western and southwestern part of Romania. Our results provide strong motivation for further studies to investigate the potential routes of exposure to AA in Romanian ccRCC patients. Although we did not find evidence for other mutational patterns that differentiate patients from higher and lower regions of incidence across our total cohort, we established a strong correlation between the number of somatic mutations in ccRCC and the age of patients at surgery. We observed that all SNV classes represent this age-associated pattern, suggesting that a general underlying process is involved. Although our observations may be due to the increased number of somatic mutations by age observed in kidney epithelial cells [32] , involvement of a cancer-associated deficiency in related cellular processes such as DNA repair cannot be excluded. Tomasetti et al. [33] have detected similar patterns in other cancers, and they argue that most somatic mutations in self-renewing tissue occur in normal cells before tumour initiation and accumulate with patient age, and most do not play a causal role in neoplasia. Further studies in which patient-matched non-tumour kidney tissue samples are analysed in addition to the tumours might contribute further understanding of these processes. Unlike in urothelial carcinoma of the upper urinary tract, the AA signature observed in Romanian ccRCC patients from our series was not associated with an increased rate of TP53 somatic mutations, a gene that is not frequently mutated in ccRCC. We observed a high frequency of somatic mutations of PBRM1 , which is the second most common mutated gene in ccRCC, among the Romanian outliers as compared with other sample pairs. However, the majority of PBRM1 mutations were not A:T>T:A transversions, implying that the higher rate of PBRM1 mutations in Romanians are not due to the AA exposure. Silencing of PBRM1 in renal cancer cell lines has shown that this protein regulates pathways involved in chromosomal instability and cell proliferation [34] . Furthermore, it has been shown that PBRM1 is required for TP53 -driven replicative senescence [35] . Given that PBRM1 is the only gene other than VHL whose mutations have been identified at the root of tumour evolution in a subgroup of ccRCCs [36] , it will be relevant to investigate the extent to which PBRM1 status is related to the AA-mutational signature or potentially other mutational patterns with additional samples in future studies. Likewise, the high rate of somatic mutations in epigenetic regulators supports the importance of chromatin remodelling/histone modification pathways in ccRCC as suggested recently [20] . In line with recent reports [19] , [20] , the PI3K/AKT/mTOR pathway was recurrently affected by somatic mutations and abnormal gene expression patterns in our series, highlighting the relevance of this signalling cascade as a therapeutic target for ccRCC. In addition, we found many components of the focal adhesion pathway among the frequently mutated genes. Besides receptor tyrosine kinase proteins that are common to focal adhesion and PI3K pathways, other members of focal adhesion were also recurrently mutated, among which COL5A3 and ARHGAP35 have recently been identified as novel ccRCC genes in a pan-cancer analysis of TCGA data [37] . COL5A3 encodes α-chain of collagen type V involved in ECM. Genes coding for other constitutes of ECM including additional collagen proteins, integrins and laminins were frequently mutated in our series. Abnormalities of ECM dynamics are common features of tumour microenvironment and play key roles in tumour formation and progression [38] , either by affecting downstream growth-promoting pathways such as ERK and PI3K signalling [39] or by contributing to angiogenesis and metastasis by influencing tumour microenvironment and tumour–stroma communication [40] . Thus, our data revealing frequent mutations in ECM components points to the likelihood of an important role of the tumour microenvironment in ccRCC. This is further supported by deregulation of cell adhesion and focal adhesion pathways observed in the gene expression profiles. Fat cadherins constitute a novel gene family identified mutated in our cohort. Fat cadherins are surface proteins that are involved in cell adhesion and modulation of signalling pathways such as Hippo and Wnt signalling [41] . Emerging evidence has shown that FAT genes are mutated in different cancers and has suggested tumour suppressor activity for these genes [42] , [43] . Together with our data, this motivates further research to dissect the mechanisms by which FAT abnormalities can contribute to cancer. Analysis of transcriptome patterns highlighted significant alterations in metabolic pathways consistent with the Warburg effect. This phenomenon is a hallmark of ccRCC [20] and emphasizes the important underlying metabolic shift in cancer cells. More generally, our study constitutes the first genome-wide characterization of the splicing alterations that are associated with renal cancer. Previous studies relied on the identification of differentially expressed exons to assess exon skipping events [44] , [45] , an approach limited to the study of a subset of splicing events. By analysing differences in exon usage and major transcript expression patterns, we showed that although major recurrent changes in splicing are rare, splicing patterns are broadly altered in ccRCC, consistent with the observation that the messenger RNA processing pathway is commonly disrupted in ccRCC [46] . Our study presents a comprehensive genomic and transcriptome characterization of ccRCC in patients from several European countries. Genome-level mutational patterns and in-depth analysis of transcriptome abnormalities reported here advance our knowledge about the molecular background of the disease, with potential clinical applications. In particular, combination of aberrant genomic and transcriptome patterns underlines focal adhesion and PI3K/mTOR pathways as recurrent molecular targets and highlights the importance of ECM and tumour microenvironment in ccRCC. Moreover, we observe strikingly different somatic mutation patterns that distinguish most of the Romanian patients from patients from other European countries included in our study. If due to AA exposure, these findings imply that the impact might be far broader than previously thought, both geographically, as none of the patients originated from known regions of endemic AAN, and for risk of developing a common cancer. Although we cannot ignore that other unknown substances could lead to similar mutational patterns, our results provide strong motivation for additional studies designed to investigate the epidemiology, biology and clinical features of ccRCCs with distinct mutational patterns in Romania, and potentially in other populations, which may lead to intervention strategies. This result also highlights the importance of including cases from multiple and diverse populations when conducting large-scale sequencing studies to determine the mutational profiles of a particular cancer. Patients and samples Patients undergoing nephrectomy for suspected renal cancer during the period December 2008 to March 2011 at St James’s University Hospital in Leeds, UK; University Hospital Motol, Prague, Czech Republic; Masaryk Memorial Cancer Institute, Brno, Czech Republic; Th. Burghele Hospital, Bucharest, Romania; and N. N. Blokhin Cancer Research Centre, Moscow, Russia, were recruited to the study after informed consent was obtained. Recruitment in Central and Eastern Europe was coordinated by the International Agency for Research on Cancer. Ethical approvals were obtained from the Leeds (East) Local Research Ethics Committee, the International Agency for Research on Cancer Ethics Committee, as well as from local ethics committee for recruiting centres in Czech Republic, Romania and Russia. All sampling and clinical data collection was undertaken according to predefined standard operating procedures following guidelines from the International Cancer Genome Consortium. The inclusion criteria for patients were ≥18 years of age, diagnosis of conventional ccRCC and no prior treatment. Exclusion criteria were a known family history of renal cancer or a defined genetic predisposition to kidney disease, such as von Hippel–Lindau disease or polycystic kidney disease, and those on haemodialysis. For patients entering the study, venous blood was obtained and the buffy coat stored for subsequent extraction of DNA. Samples of tumour and distant non-tumour cortical renal tissue were snap-frozen (with or without prior embedment in optical coherence tomography) or preserved in RNAlater as rapidly as possible following surgery (usually within 90 min). A representative haematoxylin and eosin (H&E)-stained section of formalin-fixed paraffin-embedded (FFPE) tissue was obtained for each case from the original diagnostic pathology departments and diagnostic histological details collected through standard abstract forms at each centre with grading according to the Fuhrman grading system [47] and staging using the TNM 2010 criteria [48] . Samples from 121 patients diagnosed with ccRCC were accepted into this phase of the study for analysis having passed pathological review as described below. These include samples from the Czech Republic (38 patients), Romania (14 patients), Russia (38 patients) and the UK (31 patients). WGS was undertaken for 94 cases and RNA sequencing for 91, with 36 cases analysed in both. For each case, original diagnostic H&E-stained FFPE sections were scanned using a Leica digital scanner and reviewed remotely using Slidepath software by at least two pathologists of the pathology review panel (P.H., L.E. and M.S.). For those where diagnosis of ccRCC was confirmed, frozen tissue samples (tumour and non-tumour) were processed as follows: two 5-μm sections placed on glass slides, thirty 20-μm sections placed in a tube for subsequent RNA extraction, forty 20-μm sections placed in a tube for DNA extraction and again two 5-μm sections placed on glass slides. The flanking sections at both ends of processed tumour samples were stained with H&E and also CD45, scanned and the digital images reviewed remotely by at least two pathologists of the pathology review panel (P.H., L.E. and M.S.) to confirm diagnosis and achieve a consensus assessment of grade, the presence or absence of necrosis and percentage of viable tumour cells. With one exception (due to a block selection error), all samples contained at least 70% viable tumour cells on average across the two flanking sections ( Supplementary Data 1 ). In addition, a consensus of at least 70% viable tumour cells at both ends of the blocks was achieved for all except four cases. Frozen sections from non-tumour cortical renal tissue from each patient were reviewed to confirm the absence of tumour cells and assessed for viability and the degree of inflammation. Considering the cases submitted to the study for potential entry overall (that is, to produce the 121 cases fully accepted), ~10% were rejected at the level of FFPE review as not meeting the diagnostic criteria, with a further 25% of those cases entering at frozen tissue level being rejected, largely due to insufficient viable tumour cells, that is, approximately one-third of samples considered for study entry were unsuitable. Preparation of DNA and RNA DNA samples were extracted with an Autopure (Qiagen) instrument using an automated protocol based on the salting-out method. Briefly, kidney tissue sections were manually lysed by Proteinase K digestion at a concentration of 100 μg ml −1 in the Qiagen ‘Autopure Cell Lysis solution’ overnight at 55 °C. DNA was then purified on the Autopure extractor using the manufacturer’s protocol ‘Cell Lysate Increased Spin’. DNA quality was evaluated by visualization on agarose gel of the genomic DNA or of the PCR amplification reactions of two microsatellites (D19S879 and D7S2473). For RNA extraction, tissue sections were lysed using a TissueLyzer (Qiagen) in QIAzol Lysis Reagent. After chloroform separation, the RNA was purified on a QIAcube using the miRNeasy Mini Kit following the manufacturer’s (Qiagen) instructions. The RNA purity and concentration was assessed using an Agilent 2100 Bioanalyzer and a Nanodrop spectrophotometer, respectively. Whole-genome sequencing Genomic DNA (1.5 μg) extracted from blood and tumour tissues were sheared to 300–600 bp using a Covaris E210 (Covaris, Woburn, Massachusetts, USA). Fragment libraries for a 100-bp paired-end sequencing were robotically prepared on a SPRI-TE Nucleic Acid Extractor workstation (Beckman Coulter, Inc., Fullerton, CA, USA) according to the Illumina protocol. Samples were sequenced on GAIIx and HiSeq2000 instruments (Illumina Inc., San Diego, CA, USA). RNA sequencing Indexed complementary DNA libraries were prepared from 1.5 μg of total RNA following the Illumina TRUSEQ protocol. Average size of the AMPure XP beads (Beckman Coulter, Inc.) purified PCR products was 278±9 bp. The paired-end 100 bp reads sequencing of the transcriptome was performed on pools of four cDNA libraries on a HiSeq 2000. SNP genotyping Genotyping was performed on 86 of the study blood/tumour sample pairs for which sufficient tumour DNA was available with the Human 660W-Quad v1 array (Illumina, Inc.), according to the standard manufacturer’s protocol using 200 ng genomic DNA input. Genotypes were retained on the basis of standard quality control criteria, including minor allele frequency >1%, genotype call rate >98% and lack of deviation from Hardy–Weinberg equilibrium. Analysis of WGS data We applied the FASTX-Toolkit for 3′ quality trimming using a minimum quality of Q30 and a minimum length of 32 bp. BWA backtrack was used to align each lane to GRCh37 reference genome with MT NC_012920 and the non-chromosomal supercontigs [49] . Picard ( http://picard.sourceforge.net ) was applied to adjust pair coordinates, flag duplicates and merge lanes, and GATK was used for realignment [50] . SNVs and short indels were called using SAMtools mpileup [51] with paired calling enabled and filtered with a minimum depth of 10 × . Variants were annotated using SnpEff [52] , which also includes dbNSFP and COSMIC annotations. To identify tumour-specific variants, we used a CLR (Phred log ratio of genotype likelihoods with and without pair constraint) threshold of 90 and a variant quality of 100. Putative variants were further inspected manually using Integrative Genomics Viewer visualization tool [53] . Cross-validation was made with SNP array data by extracting base calls overall and on a per lane basis for each site in the SNP array and comparing with the SNP genotypes. To identify significantly mutated genes, we used the convolution test P -value with FDR <0.2 from Genome MuSiC with region of interest built from all of RefSeq exons. CNVs were detected with DNACRD, a programme that implements an extension of the DNAcopy [54] comparative genomic hybridization array algorithm to WGS data. We only retained calls that were also detected by the control-FREEC method [55] . BreakDancer [56] and Pindel [57] were used in parallel as orthogonal techniques to identify discordant reads from Illumina paired-end sequencing data. BreakDancer was run with the following parameters: (1) minimum mapping quality of 35, (2) read-pairs within ±3 s.d. of insert size for tumour and ±2 s.d. for normal were excluded. Pindel was run according to the following parameters: (1) minimum match around breakpoint of 10 bp, (2) minimum match to reference of 50 bp and (3) minimum read mismatch rate of 0.1. For both BreakDancer and Pindel, somatic events were selected for by requiring read call support of ≥10 reads in the tumour with 0 supporting reads in the normal. Hyper- and hypo-mappability regions and microsatellite regions were discarded, and the resulting outputs were annotated according to the RefSeq (August 2010), repeat masker (open-3.30) and the Genomic Database of Structural Variants (v10) using custom scripts based on the use of the BEDTools suite [58] . BreakDancer insertion events were removed from the list of predicted structural variants, as the small insert-size selection of the library generates numerous read pairs with overlapping mate. SNVs and indels found in <10% in tumour samples or observed in control samples were excluded from further analysis. SNVs in genomic regions We classified the genome into six categories, to examine the regional distribution of SNVs. The categories were exons (CDS), 3′ UTRs, 5′ UTRs, introns, and upstream and downstream flanking regions of genes, intergenic and regions corresponding to DHS sites. Regions were extracted in BED format from the snpEff 3.4 database of hg19 for the locations of CDS, UTR and intronic regions. The upstream and downstream regions were defined as 5 kb before 5′ transcription site and 5 kb after the 3′ site. These regions are partially overlapping. DHS clusters were taken from the UCSC ‘Digital DNaseI Hypersensitivity Clusters in 74 cell types (2 reps) from ENCODE’ track. Any part of the genome not covered by the above was classified as intergenic. A genome position (base) was included in the regional analysis only if it had at least 10 × sequence coverage in all samples (calculated by the SAMtools pileup routine). Somatic mutation rates were calculated for each category and sample pair by dividing each count by the number of bases included in the category. We also calculated the normalized somatic mutation rates for each sample pair and category (the frequency of somatic mutations within the category compared with the total number of somatic mutations meeting the coverage criteria for the sample). For each category, we compared the rate with that for all other regions of the genome over all samples retained for the analysis assuming Poisson distributions and using the ‘rateratio.test’ procedure implemented in R. The data were trimmed before analysis by removing four samples that had a normalized CDS rate that was >3 s.d. from the category median across all samples. Analysis of mutational classes for outliers A statistical procedure was used to identify samples with high somatic mutation rates for one or more of the following six mutational classes: A:T>C:G, A:T>G:C, A:T>T:A, C:G>A:T, C:G>G:C and C:G>T:A. For each patient, we calculated a standardized mutation rate for each class by dividing the number of mutations in the class by the total number of mutations observed for that patient. For each of the standardized rates, we calculated a one-sided P -value for obtaining an observation as or more extreme excess using a binominal distribution with parameter θ , where θ is the median of the rate for the same class. Supplementary Fig. 3a shows the base 10 logarithm for the P -values corresponding to A:T>T:A after adjustment for multiple tests. Validation of somatic mutations We validated experimentally somatic mutations in genes that were either affected by somatic non-synonymous mutations with a frequency significantly greater than background rates ( P <0.05 from MuSiC), or mutated in at least two patients. Somatic SNVs and insertion/deletion variants were verified by pooled amplicon sequencing on Illumina MiSeq or by Sanger sequencing in the tumours and matched normal samples. PCR primers were designed to capture loci harbouring putative somatic mutations. Target loci were captured through multiplexed amplification using a Fluidigm access array system, and pools of amplicons were sequenced on MiSeq instruments. Alignments, variant extraction and quality metrics were made with BWA and in-house programmes. We considered a somatic mutation to be validated if the targeted re-sequencing confirmed the presence of the mutation in tumour and it was not found in the matched normal sample. Owing to the lack of corresponding DNA samples or unsuccessful PCR assays, we could not test further 374 out of 1,691 putative somatic non-synonymous mutations. Of the remaining 1,317 putative non-synonymous mutations, we confirmed 723 of 771 (93.7%) by Sanger sequencing and 516 of 546 (94.5%) by pooled amplicon sequencing. In total, 1,239 out of 1,317 (94.1%) of the non-synonymous mutations were validated. Analysis of RNA-seq data RNA-Seq raw reads were initially trimmed to 95 nucleotides using PRINSEQ v0.19.5 (ref. 59 ) and mapped to the reference genome using TopHat v2.0.6 (ref. 60 ). For each gene, expression counts were estimated using HTSeq v0.5.3p7 ( http://www-huber.embl.de/users/anders/HTSeq ) summarized across all its exons as annotated in Ensembl 66 using the –intersection-nonempty and –stranded=no parameters. Genes that had zero counts for ten or more samples were removed from further analysis. For the 45 matched tumour/normal samples, a paired test for differential expression was performed using edgeR [61] with tag-wise dispersion estimation and Trimmed Mean of M-values (TMM) normalization of the counts. Genes with FDR<0.01 were labelled as ‘differentially expressed’, and differentially expressed genes with median expression >1 FPKM were selected for further analysis. Gene FPKM levels were obtained by multiplying the read count for each gene with 1,000, and dividing with the total number of reads mapped to proper mate pairs to all genes and the gene length, estimated as the sum of the length of all its exons. For transcript-level analyses, we applied DEXSeq [62] to identify those genes for which at least one of the exons is differentially used between normal and tumour in the 45 matched samples. Relative abundances for annotated transcripts were obtained using MISO [63] . Transcript FPKMs were then obtained by multiplying those relative abundances with the corresponding gene FPKMs. Based on those quantifications, we identified the most abundant transcript within each gene, referred to as ‘major transcript’. The ‘major transcript dominance’ was calculated as the ratio of transcript FPKMs for the second and first most abundant transcripts for each gene. We then compared for each patient the number of genes with a different dominant transcript in the matched normal and tumour samples using a McNemar’s test, and for each major transcript in each gene we compared its dominance values in all normal against all tumour samples with a Wilcoxon test. Controlling for multiple testing was done with the Benjamini–Hochberg FDR procedure. A patient was said to exhibit a ‘switch event’ for a gene when we observed a different major transcript in the matched tumour and normal sample. Such events were further classified as either twofold or fivefold dominant if the major transcript dominance from both the tumour and normal samples exceeded this threshold. Splicing variability was calculated with the methods provided in Gonzàlez-Porta et al. [64] Identification of fusion genes Fusion genes were identified by complementary approaches. The first, implemented in deFuse [65] , identifies clusters of discordant paired-end alignments, which inform split read alignment, while the other, implemented in FusionMap [34] , searches for chimeric transcripts by identifying split reads. Putative fusion events obtained from FusionMap with the number of supporting split reads >3, or obtained with deFuse with number of spanning reads >5 and split reads >3 were retained for further analysis. The list of potential chimeric genes obtained from these putative events was further filtered by removing instances when similar patterns were found in the normal samples from study, normal samples from 462 healthy individuals provided by the Geuvadis consortium [66] and 16 normal tissues samples (Illumina Body Map, ENA: ERP000546). Subsequently, to reduce the number of false-positive chimeras, we removed mitochondrial, ribosomal genes, pseudogenes, homologous fusion partner genes, fusion events overlapping with repetitive regions and naturally occurring read-through transcripts annotated at the AceView database [67] . Finally, we examined the remaining putative fusion events with the Integrative Genomics Viewer browser [53] and pairoscope ( http://pairoscope.sourceforge.net/ ), and those that were supported by visualization were subjected to validation by reverse transcription–PCR. For validated fusion events, the open reading frame was calculated by using the frame column for each exon in the ensembl GTF file as described in ref. 65 . Protein domains were classified by ‘retained’, ‘lost’ or ‘truncated’ by extracting InterPro [68] domains of the partner genes from Ensembl via the Ensembl API ( http://www.ensembl.org/ ) and further assessing the genomic domain locations relative to the breakpoints. Gene list enrichment analysis was performed with ToppGene Suite [69] . The ideograms, coverage plots and the gene models of the fusion partner genes were drawn with the R package ggbio [70] . Validation of fusion events Fusion mRNA transcript validation experiments were performed for 16 putative fusion transcripts corresponding to 12 fusion genes identified from RNA-Seq data analysis in 17 tumour samples. For each fusion transcript, different PCR primer pairs were designed with Primer 3 ( http://frodo.wi.mit.edu/ ) using the default setting values except for the product size parameter where the minimum accepted length was reduced to 70 bp. Primer sequences are listed in Supplementary Data 18 . One microgram of tumoural and of their corresponding peritumoural total RNA, as well as of one commercial kidney sample were reverse transcribed using Superscript III (Invitrogen) and oligo(dT) primers according to the manufacturer’s instructions. Five microlitres of the cDNA solution corresponding to 5 ng of total RNA was used for PCR experiments in a final volume of 60 μl. Final concentrations of PCR mix included 1 U of HotStar DNA Taq polymerase (Qiagen), 1 × of HotStar DNA polymerase Buffer, 200 μM of each dNTPs, 200 nM of each primer and 2% of dimethylsulphoxide. The initial denaturation/activation step was performed for 15 min at 95 °C, followed by 45 cycles of 30 s denaturation at 95 °C, 30 s annealing at 60 °C and 30 s elongation at 72 °C, and a final extension step of 5 min at 72 °C in a Mastercyler Pro S (Eppendorf, Le Pecq/France). Five microlitres of PCR product was deposited with 1 × loading dye (Solis BioDyne) on a 2.5% agarose gel with 100 bp Ladder (Invitrogen) and analysed by horizontal electrophoresis in 1 × TBE buffer. For each couple of primer presenting a positive amplification in a tumoural sample, a second PCR on 5 ng of total RNA of the tumour and corresponding normal samples was performed in the same conditions to evaluate possible genomic DNA contamination. Pathway enrichment analyses Information about gene annotation to Homo sapiens (hsa) pathways was obtained from KEGG, release of December 2013, through KEGG ftp database. Total of 6,695 genes (based on entrez gene IDs) are annotated in 280 pathways according to December 2013 release. We used Fisher’s one-tail exact test to identify pathways enriched for genes affected by abnormal patterns. We controlled for multiple testing by using the Benjamini–Hochberg FDR procedure. The one-tail Fisher’s exact test for overrepresentation calculates hypergeometric probability for observing k or more genes among total K genes of each pathway based on number of total annotated genes and total queried genes. Data management and availability Clinical and sample metadata were collected and annotated using a custom-made information system KIDREP, which is based on open-source software [71] . Clinical and processed data are available from the International Cancer Genome Consortium portal. Accession codes: Raw sequence data have been deposited in the European Genome-phenome Archive (EGA), under the accession code EGAS00001000083. How to cite this article: Scelo, G. et al. Variation in genomic landscape of clear cell renal cell carcinoma across Europe. Nat. Commun. 5:5135 doi: 10.1038/ncomms6135 (2014).